Dynamic Jahn–Teller effect in the parent insulating state of the molecular superconductor Cs3C60 The 'expanded fulleride' Cs 3 C 60 is an antiferromagnetic insulator in its normal state and becomes a molecular superconductor with T c as high as 38 K under pressure. There is mounting evidence that superconductivity is not of the conventional BCS type and electron–electron interactions are essential for its explanation. Here we present evidence for the dynamic Jahn–Teller effect as the source of the dramatic change in electronic structure occurring during the transition from the metallic to the localized state. We apply infrared spectroscopy, which can detect subtle changes in the shape of the C 60 3- ion due to the Jahn–Teller distortion. The temperature dependence of the spectra in the insulating phase can be explained by the gradual transformation from two temperature-dependent solid-state conformers to a single one, typical and unique for Jahn–Teller systems. These results unequivocally establish the relevance of the dynamic Jahn–Teller effect to overcoming Hund's rule and forming a low-spin state, leading to a magnetic Mott–Jahn–Teller insulator. When superconductivity in alkali fullerides was discovered [1] , [2] , it was mostly classified as BCS type [3] . Increasing experimental [4] , [5] , [6] and theoretical [7] , [8] evidence, however, is placing these materials into the family of strongly correlated superconductors [9] . A significant step in this direction is the study of expanded trivalent fullerides. These materials are so close to the Mott localization limit that a slight change in the lattice constant can induce a transition between a superconducting and an antiferromagnetic Mott insulating ground state [10] . Cs 3 C 60 is an especially attractive member of this family because of its ordered and highly symmetric structure in both the insulating and superconducting phases [4] , [5] , [6] . Cs 3 C 60 exists in two polymorphs, one with a body-centered-based A15 structure [4] and one with face-centered cubic (fcc) structure [6] similar to K 3 C 60 (ref. 11 ) and Rb 3 C 60 (ref. 12 ). The A15 structure contains orientationally ordered fulleride ions, whereas in the fcc polymorph merohedral disorder is present. Experiments found both Cs 3 C 60 polymorphs to be Mott insulators at ambient conditions [5] , [6] , [13] , with the ions in a low-spin ( S =1/2) electronic state [5] , [13] , [14] . This low-spin state has been subject of intense discussion, where the possibility of a dynamic Jahn–Teller (JT) state was proposed [5] , [14] , putting these materials into the class of magnetic Mott–Jahn–Teller insulators. Below 46 K, A15 Cs 3 C 60 becomes antiferromagnetic [5] . The fcc polymorph also develops antiferromagnetism below 2.2 K [6] , but as a result of the fcc structure this magnetic phase is frustrated [6] , [13] . Moderate pressure turns both polymorphs into metals at high temperature [15] (up to 280 K) and superconductors at low temperature [4] , [6] , [16] . The C 60 t 1 u lowest unoccupied molecular orbital is triply degenerate, and this orbital degeneracy together with the lattice packing has a key role in stabilizing the metallic state against the Mott insulator [17] . The superconducting critical temperature ( T c ) exhibits a dome-shaped curve as a function of pressure, with maximum T c of 38 K for the A15 (ref. 4 ) and 35 K for the fcc polymorph [6] . Both the magnetic ground state and the appearance of a superconductivity dome on the phase diagram are signs of strong electron correlations, but there is no definitive understanding of the electronic and molecular structure of the resulting localized fulleride anionic species, which is key for the development of appropriate models for both the localized and nearby itinerant electronic states. The existence of the orientationally ordered and disordered polymorphs and the absence of structural transformations make this system a unique playground to study the electronic aspects of the insulator-to-superconductor transition. Approaching the problem from the molecular side, these expanded fullerides allow determination of the relative significance of the symmetry of the lattice and the molecular JT effect when a fulleride ion is placed in a solid [18] , [19] . In this paper, we employ infrared (IR) spectroscopy to address the JT effect in fcc and A15 Cs 3 C 60 as a function of temperature at ambient pressure. As in both cases the lattice possesses cubic symmetry higher than that of any possible JT distortion of the fulleride anions, the crystal field will have a secondary role to the inherent molecular interactions, which determine the distortion. We find a gradual change with temperature in the IR spectra, and explain it by the interplay of two effects: the presence of temperature-dependent solid-state conformers [20] , as observed in other JT systems [21] and the decrease of the influence of crystal field with thermal expansion. As a result, at the highest temperature, a single type of distortion, subject to pseudorotation is observed in the A15 structure. The change in the population of the different conformers results in a continuous change of the spectrum with temperature, without a structural phase transition. These spectroscopic studies thus establish the underlying molecular electronic structure of the anion in cubic fullerides, which underpins the co-operative properties of both the superconducting and insulating members of this family. IR spectra The IR spectra of both Cs 3 C 60 polymorphs ( Fig. 1 ) are markedly different from those of the metallic K 3 C 60 and Rb 3 C 60 compounds [22] . In the latter, the continuous absorption of the metallic electrons results in a strong background, which obscures the vibrational peaks. In Cs 3 C 60 , no such background is observed and the vibrational peaks are much sharper. In accordance with previous broadband spectra [5] on A15 Cs 3 C 60 , these results confirm that both Cs 3 C 60 polymorphs are insulators. This insulating state permits an analysis of the vibrational spectra, which has been impossible in other A 3 C 60 superconductors because of metallic screening. 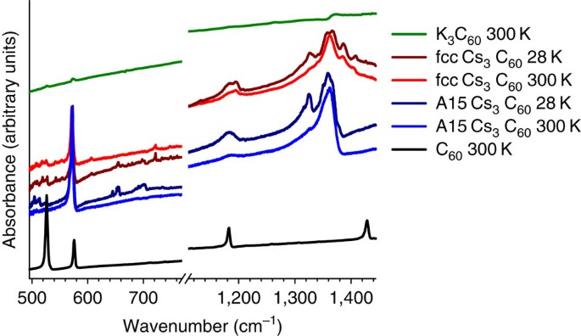Figure 1: IR spectra of A15 and fcc Cs3C60at 28 and 300 K. The energy range shown corresponds to the intramolecular vibrations. The spectra of insulating C60and metallic K3C60at 300 K are also shown for comparison. Curves have been shifted and scaled for clarity. Splitting of theT1uvibrational modes and activation of low-intensity peaks, which are silent in C60, indicate a distortion of the fulleride ion in both Cs3C60polymorphs. Figure 1: IR spectra of A15 and fcc Cs 3 C 60 at 28 and 300 K. The energy range shown corresponds to the intramolecular vibrations. The spectra of insulating C 60 and metallic K 3 C 60 at 300 K are also shown for comparison. Curves have been shifted and scaled for clarity. Splitting of the T 1 u vibrational modes and activation of low-intensity peaks, which are silent in C 60 , indicate a distortion of the fulleride ion in both Cs 3 C 60 polymorphs. Full size image The IR spectrum of neutral, undistorted (point group I h ) C 60 consists of four bands, each corresponding to a threefold-degenerate T 1 u vibration. Among these, the highest frequency T 1 u (4) mode is the most sensitive to both charge and symmetry reduction [23] . This peak is observed in both Cs 3 C 60 polymorphs around 1360 cm −1 and is split into several components. Weaker modes, which are silent in the icosahedral C 60 molecule appear in the range 600–800 cm −1 ( Table 1 ). The splitting and the activation of previously silent modes is caused by the symmetry reduction of the fulleride ion: splitting reflects the lifted degeneracy and activation of silent modes the change in selection rules. The new peaks and the splitting pattern of the T 1 u (4) peak depend on the temperature and are different in the two polymorphs. Table 1 Assignment of the newly activated weak modes in fcc and A15 Cs 3 C 60 . Full size table Temperature dependence To study the temperature dependence, we fitted the T 1 u (2) and the T 1 u (4) peaks ( Fig. 2 ) with Lorentzian functions. The T 1 u (2) vibrational mode remains unsplit in the case of the fcc Cs 3 C 60 , but appears as a doublet below about 300 K in the A15 Cs 3 C 60 . In the spectral range of the T 1 u (4) vibration, five components can be resolved at low temperature for both polymorphs. As the threefold degenerate T 1 u peak cannot split into five peaks, the silent G u (6) mode, which is found in the same frequency region [24] should also be taken into account. This mode becomes IR active upon symmetry reduction, as also seen in solid C 60 at low temperature [25] . With increasing temperature, the number of components needed for the fit gradually decreases but no distinct transition temperatures are apparent. The fits shown are for typical temperatures, where the T 1 u (4) peak can be fitted with five ( Fig. 2a,d ), four ( Fig. 2b,e ) and (in the case of A15 Cs 3 C 60 ) three components ( Fig. 2c ), respectively. The parameters of the fitted Lorentzian peaks are shown in Supplementary Figs S1,S2 . The low-intensity peaks from newly activated modes disappear at different temperatures for each mode ( Supplementary Fig. S3 ). 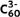Table 2 Splitting of theT1uandGurepresentations of theion in the crystal field of A15 and fcc-structured Cs3C60. No description available Figure 2: Lorentzian peak fits in the spectral region of the T 1 u (2) and the T 1 u (4) vibrational modes at selected temperatures. Fits are shown for A15 Cs 3 C 60 at ( a ) 28 K, ( b ) 180 K, ( c ) 400 K, for fcc Cs 3 C 60 at ( d ) 28 K, ( e ) 320 K. The low-temperature splitting pattern changes gradually to the one at room temperature around 80 K. In A15 Cs 3 C 60 , a further gradual transition takes place around 300 K. Full size image The simplest explanation for the observation of multiple peaks would have been that they reflect the multiphase character of the sample. This assumption is discarded after simulating the spectra of phase-pure fcc and A15 Cs 3 C 60 using the measured spectra of the fcc-rich and A15-rich samples, those of bco Cs 4 C 60 (ref. 26 ) and CsC 60 (ref. 27 ) and the known compositions of the samples. None of the additional features in Fig. 2 consistent with symmetry lowering disappears after subtracting the spectra of the known phases with the appropriate scaling factors ( Supplementary Fig. S4 ). Thus, the splitting and the activated modes are indeed signs of symmetry reduction. A prerequisite for the observation of symmetry reduction is that the molecules are not rotating. Therefore, the rotation of the fulleride ions can be considered as static on the 10 −11 s timescale of the IR measurement in both Cs 3 C 60 polymorphs, in accordance with structural data [5] , [6] . Reduction of symmetry can occur via two mechanisms and it has been ambiguous which is the dominant one in the fullerides: the crystal field shaping the molecule to its own symmetry or the molecular JT effect resulting in a symmetry reduction independent of the environment. The most important interaction in fulleride solids with large cations is the cation-fulleride ion repulsion [28] . In the A 4 C 60 salts (A=K, Rb, Cs) [26] at low temperature, steric crowding and symmetry effects cause the molecular symmetry to conform to the crystalline environment imposed by the space group (orthorhombic for Cs 4 C 60 , tetragonal for the other two) and to adopt a static D 2 h distortion, which is the largest common subgroup of the I h point group and the space groups. In the present case, however, the cation distribution has higher symmetry than the molecular symmetry indicated by the spectra. To determine the splitting in the T 1 u (4) spectral region for the case when the fulleride ion is distorted only by the crystal field, the standard correlation method has been used [29] , leading to the splitting pattern listed in Table 2 after taking into account the fulleride ion site symmetry T h in A15 and O h in fcc Cs 3 C 60 and the fact that A15 Cs 3 C 60 contains two molecules per primitive unit cell, thereby allowing for in- and out-of-phase collective modes (Davydov splitting). The last column of Table 2 gives the number of IR bands originating from the C 60 T 1 u and G u modes, respectively after considering the selection rules for dipole transitions (allowed transitions are marked (IR) in the table). As the intensity of the previously silent G u -derived modes is expected to be lower than that of the T 1 u modes, the data in Table 2 predict one strong and one weak vibrational band in both cases, in contradiction with the experiment. Table 2 Splitting of the T 1 u and G u representations of the ion in the crystal field of A15 and fcc-structured Cs 3 C 60 . Full size table Having excluded the multiphase character of the sample and the crystal field as the origin of the complexity of the IR spectra, the only remaining candidate is a JT distortion of the molecular units. Fulleride ions are subject to the JT effect because the extra electrons in the threefold degenerate t 1 u orbitals couple to the eight H g vibrations of the C 60 molecule. Thus the ion is a JT system [30] . According to theory [31] , the distortion is bimodal. The most symmetric model for such a distortion is the point group D 2 h , with the three C 2 twofold axes acting as principal axes. As the D 2 h point group does not contain degenerate irreducible representations, the t 1 u orbitals are split threefold, leading to the observed S =1/2 spin state ( Fig. 3 ). 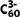Table 3 Splitting of theT1uandGurepresentations of theion on symmetry reduction from theIhto theD2hpoint group. No description available Figure 3: Molecular orbitals of molecular ions indicating the T 1 u (4) vibrations. ( a ) I h symmetry with an unsplit t 1 u molecular orbital, ( b ) D 2 h Jahn–Teller distorted molecule with threefold splitting ( b 1 u , b 2 u and b 3 u orbitals). 'Inverted Hund's rule coupling' leads to a low-spin ( S =1/2) state and the splitting of vibrational bands. Arrows represent the largest atomic displacements of the T 1 u (4) modes. The magnitude of the distortion in the molecular model is exaggerated. Full size image As the fulleride ions contain 15 twofold axes, 30 distortions are possible with the same shape but the principal axis in different directions. The molecule can be statically frozen into a single distortion or move between the differently directed distortions [20] by tunnelling or pseudorotation, leading to a dynamic JT effect. In a molecular solid built from such dynamic JT units, several scenarios are possible: free, hindered or frozen pseudorotation and in the latter case, order or disorder of the static distortion. The detection of the JT effect is complicated by the possibility of these scenarios and by the fact that the largest atomic displacement produced by the distortion is on the order of 0.04 Å (refs 32 , 33 ). In a distorted molecule, not only the electronic orbitals split but also the vibrational levels do so as well, leading to an increased number of lines in the IR spectrum. As IR spectroscopy detects the distortions through intramolecular vibrations, the contributions from molecules distorted (and oriented) in different directions add up, instead of averaging in space. To avoid time averaging, that is to detect dynamic distortions, the timescale of one spectroscopic excitation event has to be shorter than the timescale of interconversion between differently directed distortions [34] . In many cases, vibrational spectroscopy is such a method [35] , as its timescale is about 10 −11 s. Vibrational spectroscopy has identified the nature of the distortions in localized electron fullerides, which do not have the key charge. For instance, the A 4 C 60 (A=K,Rb,Cs) compounds were found to be nonmagnetic Mott–Jahn–Teller insulators [26] , [36] , [37] , [38] . The physical properties of these systems are mainly determined by the simultaneous presence of electron correlations and the JT effect, although the picture is complicated by the symmetry of the lattice. Neutron diffraction [32] in Cs 4 C 60 proved an orthorhombic lattice distortion. This distortion can in principle be explained as a cooperative JT state (D 2 h molecules ordered by translational symmetry), but as it coincides with the symmetry of the cations, it has to be regarded as a crystal field effect. NMR measurements [38] indicated a transition across a spin gap, which is evidence for JT splitting of energy levels but not diagnostic of the resulting symmetry (that is, if the splitting is two- or threefold). In this respect, vibrational spectroscopy is unique: the T 1 u vibrations have the same symmetry as the t 1 u frontier orbitals, therefore they split in an analogous fashion to the electronic orbitals. In addition, as vibrational spectroscopy detects transitions from the ground state to the vibrationally excited levels, the splitting will be seen directly if selection rules permit. This way, the static D 2 h to dynamic D 3 d or D 5 d transition was detected in the A 4 C 60 phases with the transition temperature determined by the lattice constant [26] . As mentioned above, the JT effect distorts the molecular ion into the D 2 h point group and the line splitting can be handled in a straightforward way based on simple molecular symmetry reduction [34] . The results are given in Table 3 and include three T 1 u - and three G u -derived modes. As the G u vibration is IR inactive in the neutral C 60 molecule, the peaks originating from this vibration are expected to have lower intensity, if detectable at all. These predictions agree clearly much better with the measured spectra than those in Table 2 , thus providing a clear indication of the JT character of the distortion. Table 3 Splitting of the T 1 u and G u representations of the ion on symmetry reduction from the I h to the D 2 h point group. Full size table Although the crystal field distorts the fulleride ion only slightly (from point group I h to T h , Table 2 ), it can alter the energy of the differently directed JT distortions. Distortions having principal axes parallel to the edge of the unit cell will not be equivalent to those oriented in other directions ( Fig. 4a ). The crystal field can also change the exact shape of the molecular distortion, which then influences the IR spectrum. The shape of the crystal field depends on the position of the Cs + ions surrounding the fulleride ions. This is different in the two Cs 3 C 60 polymorphs, thus accounting for the crystal structure dependence of the spectra, although the details of the exact distortions are far beyond our capacities to predict. 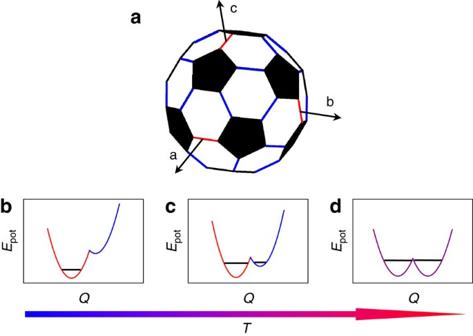Figure 4: Temperature evolution in the population of the two sets of differently directed JT distortions. (a) The hexagon–hexagon C-C 'double bonds' that the twofold axes intersect in the two kinds of distortions are labelled with blue and red on the C60molecule. The crystallographic principal axes are indicated. (b), (c) and (d) Temperature dependence of the energy relations of the potential energy minima (potential energy versus deformation coordinateQ) of the two sets of distortions. The arrow at the bottom represents increasing temperature. The filling of the energy levels is also shown. In (d) the energy minima are equivalent, thus coloured purple. The graphs are only for illustrating trends; choosing the red distortion as being lower in energy is arbitrary. Figure 4: Temperature evolution in the population of the two sets of differently directed JT distortions. ( a ) The hexagon–hexagon C-C 'double bonds' that the twofold axes intersect in the two kinds of distortions are labelled with blue and red on the C 60 molecule. The crystallographic principal axes are indicated. ( b ), ( c ) and ( d ) Temperature dependence of the energy relations of the potential energy minima (potential energy versus deformation coordinate Q ) of the two sets of distortions. The arrow at the bottom represents increasing temperature. The filling of the energy levels is also shown. In ( d ) the energy minima are equivalent, thus coloured purple. The graphs are only for illustrating trends; choosing the red distortion as being lower in energy is arbitrary. Full size image The two different possible distortions also determine the temperature evolution of the IR spectra. We use the molecular model of temperature-dependent solid-state conformers [21] , discussed thoroughly in ref. 20 . We start from two sets of distortions inequivalent in energy and follow their evolution with temperature ( Fig. 4b ). It may be possible that at low temperature, only the lower energy distortions will be realized. On heating, two effects should be taken into account. First, thermal expansion gradually reduces the strength of the crystal field (the potential energy difference between the two sets of distortions will become smaller). Second, higher energy levels become increasingly occupied ( Fig. 4c ), thus enhancing the proportion of molecules JT distorted in the direction less favoured by the crystal field. This gradual change is facilitated by the hindered pseudorotation between all possible distortions. The potential barrier decreases with temperature until there is no difference between the two sets of distortions and the molecule performs fast pseudorotation, although still somewhat hindered ( Fig. 4d ). Let us now consider the splitting found in the IR spectra. The low-temperature case with one set of distortions ( Fig. 4b ) would result in one set of peaks (3+3). The intermediate temperature with two sets of distortions ( Fig. 4c ) causes two sets of peaks. This is in contrast to the observation that the number of peaks decreases on heating. Thus above 28 K both sets of distortions are present with a continuous change in their ratio ( Fig. 4c ), giving an upper limit of 28 K≈20 cm −1 of the energy difference δ between the conformers. The fact that the population is changing smoothly with temperature proves the dynamic nature of the JT effect; it means that the barrier between conformations is low enough for continuous change of the deformation. The high-temperature case where all distortions are equivalent ( δ =0, Fig. 4d ) corresponds to one set of peaks in the IR spectrum, and thus observing fewer peaks than at intermediate temperatures. This is what is found in the measurements. There is no exact match with the predicted number of peaks (12 at low temperature to 6 at high temperature), but the number of potentially allowed peaks is such that the spectra cannot be fitted unambiguously; also the peaks assigned to the G u mode, which was silent in I h C 60 , are expected to have lower intensity. Antiferromagnetic ordering should be accompanied by ferrodistortive orbital ordering [5] and this would mean a decrease in the number of peaks in the antiferromagnetic phases [39] , [40] . In the notation of Fig. 4 , the single minimum in Fig. 4b would correspond to such a collective JT state. For the A15 polymorph, our measured temperature range reaches into the antiferromagnetic phase, but we do not observe any such effect. As the transition temperatures of orbital and spin ordering do not necessarily coincide [20] , we conclude that the static component of orbital ordering is still small at 28 K. In conclusion, we have proven the principal role of the JT effect in the parent insulating state of the expanded superconductor Cs 3 C 60 . A direct implication of our findings is that the Coulomb exchange energy, J H , which favours highest total spin and orbital angular momentum (Hund's rule) should be smaller than the Jahn–Teller interaction J JT , caused by coupling of the electrons to symmetry-lowering molecular vibrations. Their calculated magnitudes from various sources ( J H ~0.03–0.1 eV and J JT ~0.06–0.12 eV) are summarized in the review by Capone et al . [7] Although both J values are in essence independent of the lattice constant, the quantity U / W (where U is the on-site Hubbard repulsion and W the bandwidth) strongly depends on it. As under our experimental conditions both polymorphs of Cs 3 C 60 are on the localized side of the Mott transition, U/W exceeds the Mott localization limit and electron correlations are large. The localization requires U > W , so is a demonstration of the relative, rather than absolute, size of U , as W itself is also small. J H is smaller than U , but our measurements only address the competition between J H and J JT and prove the 'inverted Hund's rule coupling', that is, a low-spin state according to the JT effect ( Fig. 3 ). As the theoretical estimates of these values, quoted above, are similar in size, the present experiments are decisive in establishing the relative magnitude of these key quantities. The present results reveal that the JT effect is dynamic at all measured temperatures, but the distortion is observed as static on the timescale of the IR measurement, that is, the interconversion rate is less than 10 11 s −1 up to 400 K, the highest measured temperature. The observed distortion is dominated by the JT effect and perturbed by the crystal field to cause both a crystal structure and a temperature dependence. The crystal field results in two sets of inequivalent distortions, which become equivalent on heating as the crystal field strength decreases with lattice expansion. These features are all typical of JT systems and therefore unequivocally prove the insulating state of these correlated superconductors to be that of a magnetic Mott–Jahn–Teller insulator. The high crystal symmetry of the Cs 3 C 60 polymorphs is important in determining their highly correlated behaviour. The cubic structure does not lift the degeneracy of the t 1 u -based conduction band, and this triple degeneracy is crucial in allowing the metallic state to survive to very large values of the ratio U / W [17] . Our IR results show that the transition to the electron-correlation-driven localized state is accompanied by a loss of the degeneracy via the dynamic JT effect. As for the metallic state, we expect the degeneracy to be restored, and consequently the symmetry of the C 60 units to conform to the crystal field [35] . Such symmetry was seen in IR spectroscopy [22] and tunneling microscopy [41] experiments and further spectroscopic investigations on metallic systems are underway to test these assumptions. Sample preparation and characterization The Cs 3 C 60 samples used in this study were prepared by solution chemistry routes as described elsewhere [4] , [6] . The fcc-rich sample contained 86% fcc Cs 3 C 60 , 3% A15 Cs 3 C 60 , 7% body-centered orthorhombic (bco) Cs 4 C 60 and 4% CsC 60 , whereas the A15-rich sample contained 14% fcc Cs 3 C 60 , 71% A15 Cs 3 C 60 and 15% bco Cs 4 C 60 according to Rietveld refinements of synchrotron X-ray diffraction profiles. IR spectroscopy IR measurements were performed on a Bruker IFS 66v FTIR instrument in a flowthrough He cryostat. We measured in the temperature range 28–480 K and frequency range 500–2,000 cm −1 , with 0.25 cm −1 resolution. We found that heating promotes oxidation above 440 K for the A15, and above 350 K for the fcc polymorph even under dynamical vacuum, limiting the accessible temperature ranges for the measurements. How to cite this article: Klupp, G. et al . Dynamic Jahn–Teller effect in the parent insulating state of the molecular superconductor Cs 3 C 60 . Nat. Commun. 3:912 doi: 10.1038/ncomms1910 (2012).